Evolution of increased phenotypic diversity enhances population performance by reducing sexual harassment in damselflies The effect of evolutionary changes in traits and phenotypic/genetic diversity on ecological dynamics has received much theoretical attention; however, the mechanisms and ecological consequences are usually unknown. Female-limited colour polymorphism in damselflies is a counter-adaptation to male mating harassment, and thus, is expected to alter population dynamics through relaxing sexual conflict. Here we show the side effect of the evolution of female morph diversity on population performance (for example, population productivity and sustainability) in damselflies. Our theoretical model incorporating key features of the sexual interaction predicts that the evolution of increased phenotypic diversity will reduce overall fitness costs to females from sexual conflict, which in turn will increase productivity, density and stability of a population. Field data and mesocosm experiments support these model predictions. Our study suggests that increased phenotypic diversity can enhance population performance that can potentially reduce extinction rates and thereby influence macroevolutionary processes. Theory suggests that evolutionary changes in phenotypes should also affect population-level absolute fitness and can thus potentially alter the dynamics of both populations and communities [1] . Such effects arise because evolutionary changes in phenotypes might alter both intra- and interspecific biotic interactions, which in turn can modulate the reproductive performance of individuals and populations as a whole [2] . Natural selection is typically expected to increase the average absolute fitness and population productivity [3] . However, in some situations, natural/sexual selection might decrease population productivity and increase extinction risk, which is exemplified by cases such as the tragedy of the commons, evolutionary suicide or self-extinction [1] , [2] , [4] , [5] , [6] . It has also been suggested that certain traits (for example, sexual characters, selfishness, resistance to pathogens and self-reproduction) in particular can directly affect the population performance, including productivity, density, stability, sustainability and population fitness, which in turn might affect extinction risk [3] , [7] . Quantifying the role of evolutionary changes in phenotypes on overall population performance will increase our understanding of ecological dynamics, including demography, range expansion, community dynamics, ecosystem function and extinction risk, and elucidate how these processes in turn affect macroevolutionary dynamics [8] , [9] , [10] , [11] , [12] . However, the ecological (demographic) consequences of evolutionary changes and its underlying mechanisms have remained largely unexplored in natural populations. Few empirical studies in the past have addressed the demographic consequences of evolutionary changes. Studies on rapid evolution (that is, fast genetic change on ecological timescales of a few generations) have revealed how evolutionary changes affect ecological dynamics in laboratory settings [13] . However, the ecological consequences of long-term evolutionary changes have not been investigated in natural settings, mainly because empirical field studies are logistically very difficult to perform. An alternative approach is to investigate the spatio-temporal variation in morph frequencies of polymorphic organisms. This approach makes it possible to directly investigate the impact of gene frequency change on population dynamics. Recently, it has been suggested that polymorphisms, including plastic polyphenisms, increase population performance [14] . These kinds of phenotypic polymorphisms are generally suggested to have evolved in response to antagonism (for example,, prey–predator interaction, intraspecific resource competition and intra-/interlocus sexual conflict). The relaxation of an intraspecific antagonism might therefore be expected to enhance the productivity, evolvability, sustainability and viability of a population [8] , [11] , [14] , [15] , [16] . Such female-limited colour polymorphisms are widespread among damselflies and have been suggested to be a female adaptation to sexual harassment and hence a consequence of sexual conflict [17] , [18] . Typically, females have two or more morphs, with one ‘andromorph’ displaying a male-like colour pattern and one or two ‘gynomorph(s)’ expressing colour patterns different from males. Controlled breeding experiments have revealed that the development of female morphs is governed by a single autosomal di- or triallelic locus with expression limited to females [19] . Experimental field studies of male mating behaviours have revealed that male mate preferences for female morphs change with the frequency of female morphs, resulting in frequency-dependent male harassment [20] . Consequently, these female polymorphisms are maintained via rare-morph advantage (that is, negative frequency-dependent selection) [18] , [21] . Here, we investigated the ecological and demographic consequences of morph frequency variation in the dimorphic Ischnura senegalensis and the trimorphic I. elegans , which are two congeneric and ecologically similar damselfly species ( Fig. 1 ). To evaluate the predictions from our mathematical model, we present empirical data demonstrating how evolutionary change affects ecological dynamics in a natural population by using a combination of field observations, mesocosm experiments and the estimation of morph-specific fitness. Our results demonstrate that the evolution of female morph diversity can increase population-level performance, and may thereby influence macroevolutionary processes. 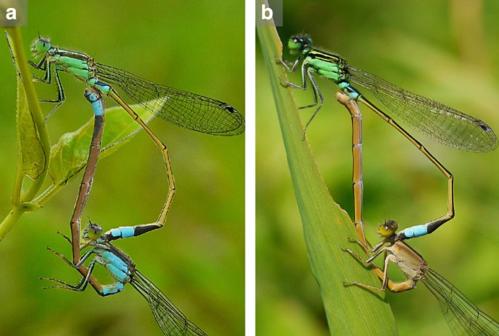Figure 1: Female colour polymorphism inI. senegalensis. (a) A male and an andromorph female. (b) A male and a gynomorph female. Female colour morphs are determined by one locus with two alleles,Dandd. Females with genotypeDDandDdare gynomorphs and with genotypeddare andromorphs. Figure 1: Female colour polymorphism in I. senegalensis . ( a ) A male and an andromorph female. ( b ) A male and a gynomorph female. Female colour morphs are determined by one locus with two alleles, D and d . Females with genotype DD and Dd are gynomorphs and with genotype dd are andromorphs. Full size image Model First, we developed a mathematical model aimed to capture the impact of male mating harassment on the fitness and population dynamics of andromorph and gynomorph females (see Methods section). Based on past empirical knowledge about the ecology and natural history of this system [18] , [21] , we explicitly incorporated female fitness and the population effects of sexual harassment by males. The strength of male mating harassment was assumed to be frequency-dependent and increases with increasing morph frequency. We also assumed a symmetric frequency dependence for the two female morphs based on previous empirical studies [20] , [21] . We therefore assumed that the effect of male mimicry on male harassment in andromorphs was negligible. Using this model, we derived quantitative predictions for the following population properties at equilibrium: the ratio of the two female morphs (morph diversity); the population density; the per capita growth rates of females of each morph; the sexual harassment risks for females of each morph and the stability of the population ( Supplementary Methods 1 ). The equilibrium ratio of the two female morphs depended on the parameters determining their intrinsic reproductive rate. In natural populations of I. senegalensis , morph frequency exhibits clinal variation [22] , [23] . Our previous study suggested that this variation in morph frequency is generated by the gene-by-environment interaction; the potential fitness of andromorph females was lower than that of gynomorph females at low latitudes, but was higher at high latitudes [22] . Thus, in our model analysis, we assumed that the intrinsic growth rate of the andromorph females b A and gynomorph females b G varies between populations at different latitudinal positions. We assumed a simple form of clinal variation: b A = B (1– L ), b G = BL , where B is a constant value and L is a value between 0 and 1 denoting the latitudinal position of the population. Under this assumption, the average of b A and b G is kept to a constant value of B /2 in all populations. To confirm that the following results are robust to deviations from this assumption, we also performed a similar analysis on the parameters b A and b G under more relaxed assumptions ( Supplementary Methods 2 and Supplementary Fig. 1 ). In Fig. 2a , we illustrate the relationship between morph diversity and the average per capita risk of sexual harassment at equilibria under various parameter sets. Each point on the curve corresponds to a parameter set at a position L , ranging from 0 to 1. The harassment risk decreased with increasing morph diversity (as the morph ratio approached 1:1). Consequently, the average per capita productivity of females, the equilibrium density of female populations and the population stability are predicted to increase with increasing female morph diversity ( Fig. 2b–d ). To confirm that our results do not depend on specific model assumptions, we performed similar analyses using a non-overlapping generation model and an individual-based model that considers a detailed life history, the behavioural property of damselflies and the genetic basis of female colour morphs. Both of these models showed similar ecological consequences ( Supplementary Methods 3 and 4 ; and Supplementary Figs 2 and 3 ). In addition, we simulated the case when there are more than two female colour morphs that allow higher female morph diversity ( Supplementary Methods 5 ). Also in this case, increased female morph diversity enhanced population performance, although this effect saturated at very high diversity ( Supplementary Fig. 4 ). 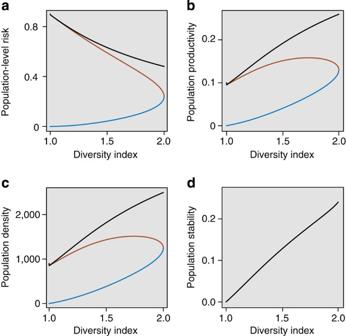Figure 2: Model predictions of the relationship between female morph diversity and population properties. Each panel shows the relationship between the diversity index of female colour morphs (black: total; blue: andromorphs; and brown gynomorphs) and the following four population properties at equilibrium under systematically varied parameter sets: (a) population-level harassment risk; (b) population productivity; (c) population density; and (d) stability of the population. Population-level harassment risk was given by (HA*FA*+HG*FG*)/(FA*+FG*), whereFA*andFG* are the equilibrium densities of andromorph and gynomorph females, respectively, andHA* andHG* are the sexual harassment risk to andromorph and gynomorph females, respectively, at the equilibrium population density. Population productivity was expressed as per capita female growth rate averaged between the two colour morphs as follows: (FA*bA(1−HA*)+FG*bG(1−HG*))/(FA*+FG*). Population stability was quantified by the maximal eigenvalue of the Jacobian matrix. The position of populationLwas varied from 0 to 1, which resulted in the variation of the per capita growth rate of the andromorphsbA(from 0 to 1) and gynomorphsbG(from 1 to 0). Other parameters were set to the following values:d=10−2,ρ=10−4,α=1,l=1, h=10−2. Figure 2: Model predictions of the relationship between female morph diversity and population properties. Each panel shows the relationship between the diversity index of female colour morphs (black: total; blue: andromorphs; and brown gynomorphs) and the following four population properties at equilibrium under systematically varied parameter sets: ( a ) population-level harassment risk; ( b ) population productivity; ( c ) population density; and ( d ) stability of the population. Population-level harassment risk was given by ( H A * F A *+ H G * F G *)/( F A *+ F G *), where F A *and F G * are the equilibrium densities of andromorph and gynomorph females, respectively, and H A * and H G * are the sexual harassment risk to andromorph and gynomorph females, respectively, at the equilibrium population density. Population productivity was expressed as per capita female growth rate averaged between the two colour morphs as follows: ( F A * b A (1− H A *)+ F G * b G (1− H G *))/( F A *+ F G *). Population stability was quantified by the maximal eigenvalue of the Jacobian matrix. The position of population L was varied from 0 to 1, which resulted in the variation of the per capita growth rate of the andromorphs b A (from 0 to 1) and gynomorphs b G (from 1 to 0). Other parameters were set to the following values: d =10 −2 , ρ =10 −4 , α =1, l =1 , h =10 −2 . Full size image Field work and mesocosm experiments Field data from multiple populations of I. senegalensis in Japan revealed that the population-level risk of male harassment decreased significantly with the morph diversity index, as predicted by our model ( Fig. 3a ). Moreover, population productivity that was estimated by female fecundity increased significantly with morph diversity ( Fig. 3b ). These observational data were experimentally confirmed in our cage experiments with I. elegans , where the mean number of mature eggs in females across morphs in populations with even morph frequencies was significantly higher than in populations with biased morph frequencies ( Fig. 3e ; and Supplementary Tables 1 and 2 ). These experimental results from our mesocosm experiments strongly suggest a higher potential growth rate in highly polymorphic (even) populations compared with more monomorphic (biased) populations. Female survival rates tended to be higher in the population with a balanced morph frequency than in populations with biased morph frequencies, although this effect was not statistically significant ( Fig. 3f ; and Supplementary Tables 3 and 4 ; Supplementary Fig. 5 ). Finally, in I. senegalensis , we also found that both the observed population density (from field censuses) and the genetically effective population sizes ( N e /habitat length) increased with morph diversity ( Fig. 3c,d ). 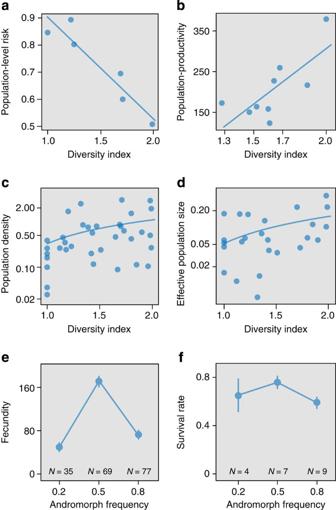Figure 3: Relationships between phenotypic diversity and population parameters in a natural population ofI. senegalensis(a–d) and mesocosm populations ofI. elegans(e,f). (a) Population-level harassment risk decreased significantly with increasing phenotypic diversity (generalized linear models (GLMs):N=9,t=−5.52,P=0.005). (b) Population productivity increased significantly with increasing phenotypic diversity (GLM:N=6,t=2.922,P=0.0223). (c) Population densities estimated on the basis of line census significantly increased with increasing diversity (GLM:N=24,t=2.227,P=0.036). (d) Standardized effective population size (Ne) also increased with significantly increasing diversity (GLM:N=35,t=2.112,P=0.042). (e) Mean fecundity across the female morphs after 1:1 morph frequency treatment was higher than that after 2:8 or 8:2 morph frequency treatments (generalized linear mixed models (GLMM):z=−3.442,P=0.0006;Supplementary Tables 1 and 2). (f) Survival rates after the mesocosm experiments did not differ significantly among frequency treatments, although the highest mean survival rate was found after 1:1 morph frequency treatment (GLMM:z=−0.6759,P=0.499;Supplementary Tables 3 and 4). Results derived from the two density treatments were pooled as the significant effects of density has not be detected for both survival rate and fecundity. All regression lines are estimated by GLM. The number of individuals (e) or trials (f) for each treatment of mesocosm experiments is shown in figures. Error bars are s.e.m. Figure 3: Relationships between phenotypic diversity and population parameters in a natural population of I. senegalensis ( a – d ) and mesocosm populations of I. elegans ( e , f ). ( a ) Population-level harassment risk decreased significantly with increasing phenotypic diversity (generalized linear models (GLMs): N =9, t =−5.52, P =0.005). ( b ) Population productivity increased significantly with increasing phenotypic diversity (GLM: N =6, t =2.922, P =0.0223). ( c ) Population densities estimated on the basis of line census significantly increased with increasing diversity (GLM: N =24, t =2.227, P =0.036). ( d ) Standardized effective population size ( N e ) also increased with significantly increasing diversity (GLM: N =35, t =2.112, P =0.042). ( e ) Mean fecundity across the female morphs after 1:1 morph frequency treatment was higher than that after 2:8 or 8:2 morph frequency treatments (generalized linear mixed models (GLMM): z =−3.442, P =0.0006; Supplementary Tables 1 and 2 ). ( f ) Survival rates after the mesocosm experiments did not differ significantly among frequency treatments, although the highest mean survival rate was found after 1:1 morph frequency treatment (GLMM: z =−0.6759, P =0.499; Supplementary Tables 3 and 4 ). Results derived from the two density treatments were pooled as the significant effects of density has not be detected for both survival rate and fecundity. All regression lines are estimated by GLM. The number of individuals ( e ) or trials ( f ) for each treatment of mesocosm experiments is shown in figures. Error bars are s.e.m. Full size image Our study indicated that populations with higher phenotypic diversity have higher per capita productivity, which is probably the result of a lower population-level mating harassment risk from males. As a consequence of this lower harassment risk, populations with more balanced morph frequencies achieve higher equilibrium population densities than more biased or monomorphic populations. Therefore, the demographic properties of our natural populations and our mesocosm experiments support the predictions of our mathematical model. Our data strongly suggest that high phenotypic diversity within populations and the evolution of polymorphisms have strong impacts on population productivity, which in turn can affect ecological dynamics. The evolution of increased diversity can therefore increase population performance including population size, population productivity and population stability. To the best of our knowledge, our study is the first to demonstrate both the underlying mechanism (male mating harassment of females and associated sexual conflict) and demographic consequences of such intraspecific evolutionary changes. The mechanism by which increased phenotypic diversity enhances population performance is connected to the risks and costs of male–female mating interactions. In these damselflies, males form a daily search image for a particular female morph and the formation of the search image depends on their previous mating experiences [20] . Hence, if a female population is monomorphic, all males will detect all females they encounter. In contrast, if the female population is polymorphic, males might therefore fail to detect a large fraction of the females they encounter due to limitations of the sensory system. As individual males develop a search image for only one type of female because of cognitive limitations. Polymorphic populations should therefore exhibit a lower level of male mating harassment compared with that in monomorphic populations. Thus, the effect of increased morph diversity on population performance is expected to be more pronounced when the population size is mainly limited by sexual conflict rather than other factors, such as resource competition (our model analysis supported this expectation: Supplementary Methods 6 ; and Supplementary Fig. 6 ). A functionally analogous process exists in predator–prey systems with frequency-dependent predation. Predators in these systems are expected to fail in detecting the non-focused prey type, suggesting that visual polymorphisms might reduce the population-level predation risk [16] , [24] . Polymorphic conditions should therefore mitigate costly interindividual or interspecific antagonistic interactions, increasing overall population performance and lowering extinction risks. The adaptive evolution of polymorphisms, including trophic polymorphisms and sexual dimorphisms, can spread various fitness costs (for example, resource limitation) or reduce the overall genetic load of a population [14] , [15] , [25] , [26] , [27] , [28] , [29] , [30] . Polymorphic systems that we studied here can illustrate evolutionary overcomes of the tragedy of the commons, in which males exploit females as common resources and thereby reduce population productivity. The positive effects of genetic diversity on the population performance might therefore be a general ecological side effect of the evolution of such polymorphisms [14] . At a higher level of biological organization, greater species diversity may increase the stability and size of the community and the productivity of ecosystems, as diversity in resource requirements may lead to more complete use of environmental resources [31] . Similarly, high intraspecific genetic diversity can enhance plant primary productivity through resource partitioning. In the present study, we have demonstrated that diversity enhances population productivity resulting in higher genetically effective population sizes ( N e ) as well as higher ecological (census) population sizes. The high effective population size when morph frequencies are balanced suggests that polymorphism increases population stability, consistent with the predictions of our model and in accordance with our empirical results. Polymorphic populations should therefore be able to exploit wider niches than monomorphic populations with a reduced risk of resource depletion, which may increase their resilience to extinction under the fluctuating environmental conditions [14] , [32] . This suggests that evolution of polymorphism can increase population fitness. In the present study, we did not consider the effect of abiotic and biotic environments of each habitat on population productivity. These can be potential confounding factors explaining the observed pattern of population performance. However, the effect of any spatial difference in biotic/abiotic environments may be mitigated in our field works, since we randomly chose all of our study populations. In addition, the predictions from the mathematical model and our simulations, both of which did not incorporate spatial difference in biotic/abiotic environments, were very consistent with our empirical data. Thus, we are convinced that such environmental variation is at most a minor factor affecting population productivity, compared with the stronger effects of intraspecific mating interactions between males and females. Also, we did not explicitly analyse the effect of demographic stochasticity. Theoretically, demographic stochasticity is suggested to lead to population extinction and/or loss of polymorphism. However, such impact may be mainly restricted only in small populations or populations with biased equilibrium morph frequency. Thus, demographic stochasticity will not change qualitatively the conclusions of this study. The understanding of the side effects of evolution on demographic dynamics has only recently gained increasing research attention [14] , [33] , [34] , [35] . Such side effects can potentially explain spatio-temporal patterns of communities and ecosystem functions [7] , [11] . In addition, changes in the sustainability of populations (that is, population fitness) can in turn influence macroevolutionary patterns including speciation and extinction rates [8] , [10] , [12] . Further studies quantifying the side effects of microevolutionary changes are required for a complete understanding of population, community and ecosystem dynamics, as well as macroevolutionary diversification. Model To investigate the relationship between the diversity of female colour morphs and the population process, we developed a mathematical model aimed to capture the dynamics of the female population. Here we describe the ecological assumptions underlying this model and present the mathematical model in more detail. We derive predictions for equilibrium morph frequency, population density and the stability of populations by considering the variation in model parameters caused by a morph-specific geographic cline in female fitness [22] , [23] . Female colour morph diversity within a population ( D ) was calculated using the Shannon species diversity index [36] : , where p i is the frequency of the female morph with the i th body colour, and m is the number of colour morphs in a population. Therefore, when there are two morphs ( m =2), D will be close to the maximum value when the frequencies of these two colour morphs are similar (that is, a 50:50 ratio). This index is useful because it can also be used when there are more than two morphs in a population. Ecological assumptions In damselflies, the per capita fecundity of females decreases with the intensity of sexual harassment by males, because females lose time for feeding and egg laying when they experience mating harassment [21] , [37] . Males search for females based on visual images of their previous mating partners; therefore, males tend to more frequently approach females of the colour morph that is most common in a population. This male sexual harassment associated with learning results in a negative frequency-dependent selection on female colour morphs [18] , [21] . Based on this empirical knowledge, we assumed that the negative effect of sexual harassment on the per capita fecundity of a female individual increases both with the male density and with the frequency of the focal colour morph [21] , [38] , [39] . For simplicity, we assumed that generations are continuous and we did not explicitly incorporate the exact genetic background underlying the female colour morphs in this mathematical model. To confirm that this simplification did not cause qualitative changes in the results, we also constructed an individual-based computer simulation model with discrete generations, assuming a di-allelic one-locus determination of female colour morphs [19] , [40] , [41] . In natural populations, the female morph frequency exhibits clinal variation, which is generated by the difference in potential fecundity between female morphs in each population [22] , [23] . Previous studies have shown that the potential fecundity of the different female morphs of I. senegalensis changes with latitude [22] . The potential fecundity of andromorph females is lower than that of gynomorph females at low latitudes, but higher at high latitudes. In our model, we assumed that the intrinsic reproductive rate of females with two colour morphs varied with the geographic position of the population. Population dynamics We assumed that the female population grows logistically. Based on the assumptions described above, the population dynamics of females with two different colour morphs are given as follows: where F A and F G denote the density of andromorphs and gynomorphs, respectively, and M is the density of males. The first terms in the right side of equations (1a,b),  are birth rate. b A and b G are the per capita reproduction rates of andromorphs and gynomorphs in the absence of male sexual harassment, respectively. H A and H G indicate the effects of male sexual harassment on the fecundities of females of the two morphs. The second terms in the right side of the equations are death rate. The parameter d is the basal death rate, and ρ /2 is the intensity of intraspecific competition. As explained above, the costs of sexual harassment, H A and H G , increase in a frequency-dependent manner. Here we assumed the following form for the risk of sexual harassment on females that is one of the simplest functions that shows frequency dependence: where α is the coefficient determining the strength of sexual harassment. The first fraction incorporates the frequency dependence caused by male learning. The parameter l indicates the intensity of learning by males, which in turn determines the intensity of the frequency dependence of sexual harassment. The second fraction considers the increase in sexual harassment on female individuals with an increase in male density. Because the number of males with which individual females encounters is limited by the length of the mating period, the risk of sexual harassment was assumed to saturate under high male density. The parameter h is the saturation rate of sexual harassment on a female with an increase in male density. In the following analysis, we assumed that the sex ratio is 1:1, and thus, the male density M is equal to the female density ( F A + F G ). By substituting M by ( F A + F G ), equations (1a,b),  will become: To predict the equilibria in populations with different female morph diversities, we systematically varied the parameter values. As described above, much of the variation in female morph frequencies between different populations is generated by the latitudinal cline in the potential fecundity of each morph. Therefore, we assumed that b A and b G varies between latitudes. Assuming that the average of b A and b G is equal to a constant value B /2 in all populations, b A and b G were assumed to be given as follows: b A = B (1– L ), b G = BL , where L is an number between 0 and 1 that denotes the latitudinal position of the population. Other parameter values used in the model analysis are summarized in Supplementary Table 5 . Although this assumption is useful for the analysis, we were aware that the average of b A and b G may not always be constant between all populations in nature. Therefore, we also analysed the equilibrium of the model under a more general assumption that b A and b G randomly varied in each population from the basal value ( Supplementary Methods 1 ; Supplementary Fig. 1 ). Results from the models using these two different assumptions were qualitatively similar, suggesting that the relationship between female morph diversity and population properties is not sensitive to the detail of the model assumptions. Study sites and morph frequencies Morph frequencies in both I. senegalensis and I. elegans geographically vary, with higher andromorph frequency at higher latitudes [22] , [23] , [42] . At least for I. senegalensis , this cline in morph frequency is established by the combination of negative frequency-dependent selection, which is derived from frequency-dependent sexual harassment, and genotype-by-environment interaction set by different temperature conditions along the north–south cline [22] , [23] . Because andromorphs have slightly higher fitness than gynomorphs at lower latitudes but lower fitness at higher latitudes; therefore, the equilibrium frequency changes with latitude. For I. senegalensis , 37 populations with different morph frequencies were studied in Japan between the years 2009 and 2011. A population of I. elegans was studied in Sweden in the summer of 2012. The Swedish population provided a more extreme andromorph-biased population than could be found in I. senegalensis in Japan, where all populations are gynomorph-biased and andromorphs are the minority morph. In all of our study populations, the morph frequency was estimated by line census. The number of males and females of each morph and female reproductive status (mature or immature) were recorded during field transects (see Supplementary Information for details of the study sites). Unlike I. senegalensis , I. elegans occurs in three female morphs: one andromorph and two gynomorphs ( infuscans and infuscans-obsoleta ), but the least common morph ( infuscans-obsoleta ) was not found in the study population on the day of the experiment. When a population was sampled more than once (at different times during the spring generation), the mean of the replicates was used as the morph frequency. Population-level harassment risk To estimate population-level harassment risk, presentation tests were performed in six local I. senegalensis populations. Females of each morph were presented to mature males, and behaviour of the males (sexual or non-sexual) was recorded. To obtain data from an extremely andromorph-biased population, the same procedure was conducted in one population of I. elegans in Sweden, where andromorph females are typically in the majority. Population-level harassment risks were defined as p × R A + q × R G , where p and q are the proportions of andromorphs and gynomorphs in sexually mature females ( p + q =1), respectively, and R A and R G are the proportions of mature males that show sexual behaviour towards the presented andromorphs and gynomorphs, respectively. Population productivity Population productivity was estimated in nine geographically isolated local populations of I. senegalensis . The individual absolute fitness w of each morph was estimated as the difference in the average number of eggs loaded before and after their daily oviposition activity [37] . Population productivity was defined as p × w A + q × w G , where w A and w G are the estimated individual absolute fitness in andromorphs and gynomorphs, respectively. To experimentally and more directly investigate the effect of colour morph frequency on population fitness, we performed a mesocosm experiment in outdoor cages with different morph frequencies of I. elegans . Population fitness was estimated in experimentally manipulated populations in the outdoor cages (3 × 3 × 3 m 3 ) at the Stensoffa ecological field station, belonging to Lund University and located 20 km east of Lund. Individuals of I. elegans were collected from populations in the area around Lund in June 2012. Field-caught males and females were released into housing cages, which contained small artificial ponds and natural vegetation. Small insects naturally entered through the mesh (2 × 4 mm) of the cages. Females generally mated during the morning and were often observed laying eggs in the artificial ponds in the afternoon. Field-caught individuals of both sexes were held in the housing cages for at least 3 days to acclimatize to the cage environment and to reach sexual maturation. To control the mating experience of males and to avoid using virgin females and immature individuals in the experiments, mating pairs identified in the housing cages were transported to the experimental cages. The frequency of the two female morphs (20, 50 and 80% for the andromorphs) and the total population density (20 individuals for low density, 40 individuals for high density) in the experimental cages were manipulated while maintaining a 1:1 sex ratio. To simplify the experiment, we used the infuscans morph instead of the infuscans-obsoleta morph (which was the less common gynomorph in the study region) as the single gynomorph. After 2 days, surviving females were collected and the number of mature eggs loaded (fecundity) was recorded. Population density Field population densities were calculated based on the total number of individuals in and the length of the census line ( Supplementary Table 6 ). For molecular analyses, adult individuals of I. senegalensis were collected from 29 of the 36 populations, for which morph frequencies were measured. The thorax of each captured individual was immediately preserved in 2 ml absolute ethanol and stored at −20 °C until DNA extraction. Both males and females were used for the genetic analyses. The average number of individuals used for microsatellite analysis in each population was 18.7±5.71 (±s.d. ; see Supplementary Table 6 for details on the number of specimens examined). The thorax muscles of individual damselflies were incubated for 3 h in extraction buffer (0.1 M Tris, pH 8.0, 10 mM EDTA and 0.2 mg ml −1 proteinase K) at 50 °C, and total genomic DNA was purified using the Wizard Genomic DNA Purification Kit (Promega). Alleles at six previously developed microsatellite loci (I002, I015, I053, I058, I034 and I210; refs 23 , 43 ) were amplified by polymerase chain reaction (PCR). PCR products were separated and alleles were detected using an ABI 3130 sequencer. GeneMapper 3.0 (Applied Biosystems) was used to determine the genotypes of the individuals for the neutral loci. All loci were tested for Hardy–Weinberg equilibrium and for linkage disequilibrium using GENEPOP version 3.4 and operating a Markov chain approximation with 10,000 iterations in 1,000 steps. The effective population size, N e , was estimated using NeEstimator [44] , [45] . N e for each population was standardized based on the length of each habitat (the vegetative shoreline length of a pond; see Supplementary Table 6 ). Statistical analyses All statistical analyses were performed using R version 3.0.1 (ref. 46 ). The relationships between morph diversity and harassment risk, population-level absolute fitness and population size were analysed using generalized linear models assuming Poisson or Gaussian distribution. The effects of morph frequency and population density on each population parameter (fitness and survival rate) in the mesocosm experiments were analysed using generalized linear mixed models in the glmmML package for R, assuming Poisson or binomial distribution and with experimental replicate (cage session) as a random factor and density treatment, frequency treatment and female morph as categorical and fixed factors. How to cite this article: Takahashi, Y. et al. Evolution of increased phenotypic diversity enhances population performance by reducing sexual harassment in damselflies. Nat. Commun. 5:4468 doi: 10.1038/ncomms5468 (2014).